Genome biology of the paleotetraploid perennial biomass cropMiscanthus Miscanthus is a perennial wild grass that is of global importance for paper production, roofing, horticultural plantings, and an emerging highly productive temperate biomass crop. We report a chromosome-scale assembly of the paleotetraploid M. sinensis genome, providing a resource for Miscanthus that links its chromosomes to the related diploid Sorghum and complex polyploid sugarcanes. The asymmetric distribution of transposons across the two homoeologous subgenomes proves Miscanthus paleo-allotetraploidy and identifies several balanced reciprocal homoeologous exchanges. Analysis of M. sinensis and M. sacchariflorus populations demonstrates extensive interspecific admixture and hybridization, and documents the origin of the highly productive triploid bioenergy crop M. × giganteus . Transcriptional profiling of leaves, stem, and rhizomes over growing seasons provides insight into rhizome development and nutrient recycling, processes critical for sustainable biomass accumulation in a perennial temperate grass. The Miscanthus genome expands the power of comparative genomics to understand traits of importance to Andropogoneae grasses. In addition to its historical roles in paper production and as ornamentals, varieties of the wild grass Miscanthus can produce high yields of harvestable vegetative biomass while maintaining and potentially increasing soil carbon [1] . These features, enabled by C4 photosynthesis, perenniality, and related high efficiencies of light, nutrient, and water use, make Miscanthus and its close relatives (including sugarcanes and energy canes) promising candidates for economically feasible and sustainable bioenergy crops [2] , [3] , [4] . Continued genetic improvement of bioenergy feedstocks is needed to enhance productivity and ensure that these crops remain robust in the face of ongoing biotic and abiotic stresses. This is particularly true for perennial grasses, where the advantages in economic and environmental sustainability relative to annuals depend on the longevity of the crop once established. Although perennial crops have tremendous potential for maximizing agricultural yields and minimizing environmental impacts, our knowledge of their biology and ability to manipulate their genetics lags well behind that in annual crops [5] . A key limitation to the genetic improvement of perennial bioenergy grasses is the complexity of their genomes, which hinders the application of modern breeding approaches [6] . Miscanthus sinensis is a genetic diploid (2 n = 38) with a genome size of 1C = 2.4–2.6 Gb [7] ; the related M. sacchariflorus occurs in both diploid (2 n = 38) and tetraploid (2 n = 76) forms. The n = 19 monoploid chromosome set of Miscanthus arose by ancient doubling of a sorghum-like n = 10 ancestor, with a single chromosomal fusion [8] , [9] , [10] . Interspecific hybrids of Miscanthus form readily, even between individuals of different ploidy [11] , [12] . Indeed, the predominant commercially grown miscanthus bioenergy variety is the high-yielding, sterile, asexually propagated triploid hybrid M. × giganteus “Illinois” (3 n = 57). It is a clone of the taxonomic-type specimen, holotypus 1993–1780 Kew [13] , [14] . Polyploidy is also common within the Saccharum complex, a group of closely related and highly productive perennial C4 grass species in the subtribe Saccharinae that includes sugarcanes ( Saccharum spp.) and miscanthus. Intergeneric hybrid “miscanes” have been made by crossing miscanthus with hybrid sugarcanes [15] , suggesting that natural genetic variation in these two genera could be combined in order to blend desirable traits (e.g., cold tolerance and disease resistance). Here we establish miscanthus as a genomic model for perenniality and polyploidy, and develop a foundation for genomic variation that will enable the future improvement of perennial biomass crops. We describe a draft chromosome-scale genome sequence for M. sinensis , prove that miscanthus is a paleo-allotetraploid by analyzing the distribution of transposable elements across its genome, and establish the timing of key evolutionary events. By mRNA sequencing, we identify genes preferentially expressed in rhizomes, stems, and leaves, and explore the unique transcriptional dynamics of nutrient mobilization in this rhizomatous perennial grass. Unlike most perennial Andropogoneae, which are restricted to tropical or subtropical regions, the Miscanthus genus comprises species that naturally range from tropical to subarctic regions. Genomic analysis of 18 miscanthus accessions sequenced for this study, in addition to reduced representation genotyping of over 2000 accessions collected in the wild from east Asia, reveals extensive population structure and interspecific introgression, which further contributes to the genomic diversity of the genus Miscanthus . Genome sequence and organization We assembled the M. sinensis genome into n = 19 chromosomes by combining short-read whole-genome shotgun (WGS) and fosmid-end data with in vitro [16] and in vivo [17] chromatin proximity libraries (Supplementary Fig. 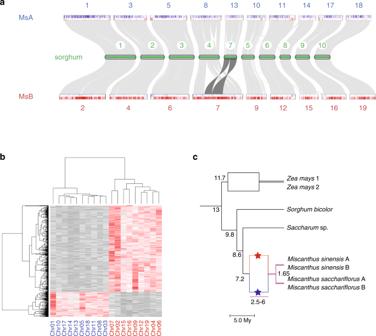Fig. 1: Allotetraploidy in miscanthus. aSyntenic relationships between sorghum andM. sinensissubgenomes MsA and MsB. Distribution of subgenome-specific 13-mer sequences (blue for MsA, red for MsB) is shown for eachM. sinensischromosome (see text and Supplementary Note7.1).bClustering of counts of 13-mers that differentiate homeologous chromosomes enables the consistent partitioning of the genome into two subgenomes. Blue chromosome names correspond to the A subgenome, red chromosome names correspond to the B subgenome.cTimetree of Andropogoneae showing the timeline of allotetraploidy in theMiscanthuslineage, with divergence and hybridization times of the A and B progenitors estimated from sequence comparisons (Supplementary Note8). Source Data underlying Fig. 1b are provided as a Source Data file. 1 , Supplementary Table 1 , and Supplementary Notes 1 , 2 ). The reference accession is the previously characterized [8] doubled haploid DH1, which as expected is homozygous throughout. 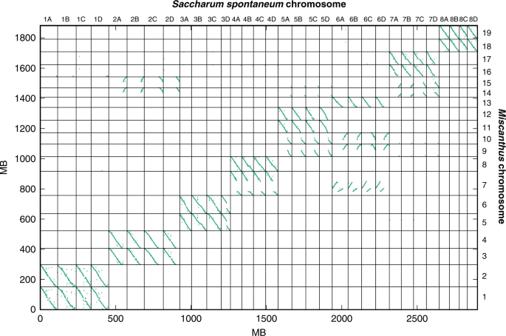Fig. 2:Miscanthus–Saccharumsynteny. Dotplot showing co-orthologs betweenMiscanthus sinensisandSaccharum spontaneum. All syntenic genes with c score ≥ 0.7 are shown using the mcscan ortholog algorithm. Note the 2:4 ratio of miscanthus:sugarcane chromosome segments. Source Data are provided as a Source Data file. The genome assembly anchors 1.68 Gb of contigs to chromosomes, with a contig N50 length of 33.1 kb and pre-HiC scaffolding N50 length of 190 kb (Supplementary Table 2 ). An additional 0.20 Gb of contig sequence in scaffolds is not yet placed on linkage groups; highly repetitive sequences are problematic and missing from the assembly (Supplementary Fig. 1b ). We validated the assembly at chromosome scale by comparison with an integrated genetic map with 4298 assignable markers (Supplementary Note 3 ). We predicted the structure of 67,967 protein-coding genes based on several lines of evidence, including homology with other grasses and deep transcriptome data for miscanthus and sugarcane [18] . These predicted genes account for an estimated 98% of protein-coding genes, with 94% assigned to a chromosomal position (Supplementary Tables 3 – 5 , Supplementary Fig. 5 , and Supplementary Note 4 ). These genes are embedded within a sea of transposable element relicts and other repetitive sequences, which account for 72.4% of the M. sinensis genome assembly. The most common class of assembled transposons are gypsy long-terminal-repeat (LTR) retrotransposons (Supplementary Table 6 and Supplementary Note 5 ). The paleotetraploidy of miscanthus is evident at the sequence level, since each sorghum chromosome aligns to a pair of M. sinensis chromosomes, after accounting for the chromosome fusion of ancestral sorghum 4- and 7-like chromosomes [8] that reduces the karyotype from n = 20 to n = 19 (Fig. 1a ). As expected from earlier genetic maps [8] , [9] , [10] (Supplementary Fig. 3 ), the miscanthus and sorghum genomes show extensive 2:1 conserved collinear synteny (Fig. 1a and Supplementary Fig. 4a ), consistent with a whole-genome duplication in the Miscanthus lineage. While it has been suggested [19] that this duplication could be shared with sugarcane, comparison of M. sinensis and S. spontaneum [20] genomes shows that the duplications in the two lineages are distinct (Supplementary Note 7 and Fig. 2 ). Although the doubled genome and disomic genetics of miscanthus is suggestive of an allotetraploid history, neither a mechanism nor timing for paleotetraploidy has been described, in part due to the absence of known diploid progenitor lineages. We address this further below. Fig. 1: Allotetraploidy in miscanthus. a Syntenic relationships between sorghum and M. sinensis subgenomes MsA and MsB. Distribution of subgenome-specific 13-mer sequences (blue for MsA, red for MsB) is shown for each M. sinensis chromosome (see text and Supplementary Note 7.1 ). b Clustering of counts of 13-mers that differentiate homeologous chromosomes enables the consistent partitioning of the genome into two subgenomes. Blue chromosome names correspond to the A subgenome, red chromosome names correspond to the B subgenome. c Timetree of Andropogoneae showing the timeline of allotetraploidy in the Miscanthus lineage, with divergence and hybridization times of the A and B progenitors estimated from sequence comparisons (Supplementary Note 8 ). Source Data underlying Fig. 1b are provided as a Source Data file. Full size image Fig. 2: Miscanthus – Saccharum synteny. Dotplot showing co-orthologs between Miscanthus sinensis and Saccharum spontaneum . All syntenic genes with c score ≥ 0.7 are shown using the mcscan ortholog algorithm. Note the 2:4 ratio of miscanthus:sugarcane chromosome segments. Source Data are provided as a Source Data file. Full size image Regarding the more than twofold difference in bulk genome size between sorghum and miscanthus, we find that lengths of coding sequence and introns are generally similar (Supplementary Fig. 4b, c ), with overall differences arising from increased intergenic spacing in miscanthus due to transposon insertion, as well as by the expansion of repetitive pericentromeric regions, which are only partially captured in the assembly (Supplementary Fig. 4b ). The chromatin conformation contact map (Supplementary Fig. 2a ) exhibits an enrichment of centromeric and telomeric contacts, respectively, consistent with the interphase nuclear “Rabl” conformation as seen in the barley genome [21] . We identified locally interacting chromosomal compartments (Supplementary Fig. 2b and Supplementary Note 2 ) for which A compartments have a higher gene density and B compartments have lower gene density (one-sided t -test p value < 2.2 × 10 −16 ) and tend to occur predominantly in the pericentromeric region, as observed in other plants [22] . Allotetraploid origin of Miscanthus An allotetraploid (i.e., hybrid) origin for a paleotetraploid species is commonly demonstrated by showing that one set of its chromosomes (a subgenome) is more closely related to some diploid lineages to the exclusion of others [23] . Because there are no known candidates for the diploid progenitors of tetraploid miscanthus, this approach cannot be used here. Instead, we used a new method that relies on the chromosomal distribution of repetitive elements, which can provide robust markers for subgenome ancestry [24] . We sought repetitive sequences whose presence is enriched on one member of each homeologous chromosome pair (Supplementary Note 6 ). Such sequences are definitive markers of allotetraploidy, and occur as relicts of repetitive elements that were active in only one of the two diploid progenitors prior to hybridization and genome doubling [24] . Importantly, the method does not require access to or even knowledge of living representatives of the progenitor lineages. We found 1187 13-bp sequences (13-mers) whose pairwise enrichment pattern consistently partitions homeologous chromosome pairs between distinct A and B subgenomes (Fig. 1a, b ). This observation establishes the past existence of distinct A and B progenitor lineages (which remained separate for millions of years, see below), and the allotetraploid origin of miscanthus. Although we can use these markers to assign each miscanthus chromosome in bulk to the A or B subgenome, we find evidence for the balanced reciprocal exchange of distal segments between homeologous chromosomes such that dosage remains intact (e.g., the ends of chromosomes 5–6, 11–12, and 16–17; Figs. 1 a, 3a , Supplementary Fig. 6 , and Supplementary Note 6 ). Based on consistency with our dense genetic map, these are clearly bona fide homeologous exchanges rather than misassemblies. The observed distal reciprocal exchanges likely occurred either by mitotic recombination in the vegetative tissue of an AB F1 hybrid founder prior to genome doubling, or by aberrant homeologous recombination after allotetraploidy. The concentration of these exchanges toward the ends of chromosomes is consistent with the proximity of these regions in a telomeric bouquet conformation. The maintenance of discrete A/B patterns of diagnostic 13-mers in these distal segments implies that these exchanges occurred by single crossover events rather than recurring recombination throughout the distal regions of the chromosomes, which would blur the distinctive A/B 13-mer signature. Fig. 3: Post-allotetraploidy reciprocal exchanges. a Example of a chromosome pair without reciprocal exchange (chr01–chr02), and two chromosome pairs with distal reciprocal exchanges (chr05–chr06 and chr11–chr12). Red and blue dots represent occurrences of subgenome-specific 13-mers. Black bars identify A and B ancestry inferred from a Hidden Markov Model (Supplementary Note 7.2 ). b Relative expression of homeologous gene pairs. Across tissues and seasonal sampling times, there is a 3.8% median bias toward the expression of the B member of the pair. c Homeologous gene pairs within reciprocally exchanged regions show the expression bias of their ancestral location. Source Data underlying Fig. 3b, c are provided in the Source Data file. Full size image Discrete homeologous exchanges are often observed in newly formed allotetraploids and are thought to occur in response to a new meiotic environment [25] . In studies of other polyploids, homeologous replacements that alter the balance between A and B alleles are common; when such variants are segregating in a population, the resulting genetic variation can underlie quantitative trait loci [26] , [27] . In contrast to these studies, however, in Miscanthus , we find (1) predominantly balanced reciprocal exchanges that alter chromosomal linkage, but do not change A/B dosage, and (2) no evidence that these segmental exchanges are segregating in our sequenced samples, suggesting that the reciprocal homeologous exchanges are the result of ancient events that have become fixed in Miscanthus (and therefore cannot be causal for any phenotypic variation in the genus) (Supplementary Note 6 )). In addition to these long fixed reciprocal exchanges, there are several shorter internal homeologous segments (Supplementary Note 6 ) that could correspond to nonreciprocal or recurrent exchange. These segments will be interesting to study further. From the identification of distinct A and B subgenomes, we see that the sorghum-7 and -4-like chromosomes that fused [8] to form miscanthus chromosome 7 were both derived from the B progenitor. While it is possible that the fusion occurred in the B progenitor itself prior to hybridization, the absence of other Saccharinae with n = 9 chromosomes, and the likelihood of chromosome instability in the aftermath of allotetraploidization, suggests that the fusion occurred after allohybridization. The timeline of paleotetraploidy in miscanthus can be established through inter- and intra-subgenome comparisons (Fig. 1c and Supplementary Note 7 ). We estimate that the A and B progenitors diverged from their common ancestor ~7.2 Mya (million years ago), based on the synonymous differences between homeologous protein-coding genes (Supplementary Fig. 7 ). After this divergence but before hybridization, the two (now likely extinct) progenitors evolved independently; evidence of their species-specific transposable element activity appears in the contemporary Miscanthus genome as subgenome-specific repeats [24] . Consistent with this hypothesis, we find several LTR-retrotransposon families within only one of the two subgenomes, and estimate that they were actively inserting during the period ~2.5–6 Mya (Supplementary Note 7 ). In contrast, transposon activity after the allotetraploidy event should be distributed across the entire Miscanthus genome without regard to subgenomes. Also, consistent with this picture, we find a burst of transposon activity that is not subgenome-specific starting ~2.5 Mya, which serves as our best estimate for the allotetraploid origin of Miscanthus (Supplementary Note 7 and Supplementary Fig. 7c ). Finally, the interfertile sister species M. sinensis and M. sacchariflorus diverged ~1.65 Mya (Fig. 1c ), consistent with speciation occurring after allotetraploidy. Chromosome-level comparisons of repetitive elements and protein sequences confirm that the polyploidies of Miscanthus and sugarcane occurred independently (Supplementary Note 7 ). Common hallmarks of allopolyploidy are asymmetric gene loss (or conversely, retention) and biased gene expression between subgenomes, which are both thought to arise from epigenetic asymmetries in the aftermath of allohybridization [28] , [29] . Comparing miscanthus and sorghum genes, we find that ~29% of sorghum genes have been lost on one of two subgenomes; conversely, ~71% have co-orthologs on both subgenomes (Supplementary Note 6 ). Gene retention in M. sinensis shows a small but statistically significant bias toward the B subgenome (87.1% genes retained on B vs. 83.9% on A, Supplementary Table 7 ; Fisher’s exact p value, two-sided = 1.2 × 10 −9 ). The level of homeologous gene retention in M. sinensis is nearly twice that of maize (71% vs. 36%), presumably because the miscanthus allotetraploidy is more recent. The subgenome retention bias in Miscanthus is also smaller than in maize [28] (80.6% in maize 1 vs. 55.4% in maize 2), which may reflect differences in the degree of genomic differentiation between maize versus Miscanthus progenitors prior to hybridization. Similarly, for retained homeolog pairs, we find a weak but significant expression bias (median B/A expression ratio 1.038, without strong variation across tissues or season, Fig. 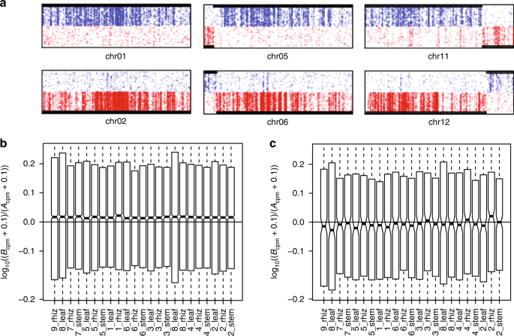Fig. 3: Post-allotetraploidy reciprocal exchanges. aExample of a chromosome pair without reciprocal exchange (chr01–chr02), and two chromosome pairs with distal reciprocal exchanges (chr05–chr06 and chr11–chr12). Red and blue dots represent occurrences of subgenome-specific 13-mers. Black bars identify A and B ancestry inferred from a Hidden Markov Model (Supplementary Note7.2).bRelative expression of homeologous gene pairs. Across tissues and seasonal sampling times, there is a 3.8% median bias toward the expression of the B member of the pair.cHomeologous gene pairs within reciprocally exchanged regions show the expression bias of their ancestral location. Source Data underlying Fig. 3b, c are provided in the Source Data file. 3b ). Although most pairs of homeologous genes have similar expression levels, there are ~10% more pairs with higher B-subgenome expression than vice versa (Supplementary Table 8 ). This is again notably weaker than the expression bias in maize [28] . Interestingly, genes in regions of homeologous exchange show (on average) the bias of their source subgenome (Supplementary Note 8 and Fig. 3c ), indicating that subgenome expression bias arises from local effects and/or became fixed early in the allotetraploid evolution. This observation is consistent with experiments that show rapid development of subgenome bias in neoallopolyploids [25] , [30] , [31] . The weaker subgenome expression and retention bias seen in the more recent miscanthus allotetraploidy versus the older maize suggests that these effects may become amplified over time, and may also be influenced by the relative genomic divergence of progenitors. Seasonal dynamics of gene expression As a rhizomatous perennial, miscanthus provides a model for studying the biology of rhizomes, which are modified underground stems that enable temperate perennial grasses to overwinter by their capacity to (1) store nitrogen, carbon, and other nutrients from senescing leaves and stems, and (2) mobilize these reserves in the spring to feed new vegetative growth. Amino acids, particularly asparagine with its high N:C ratio, are the primary form of nitrogen cycled among plant tissues [32] . Monitoring free asparagine concentrations (Fig. 4a ) from stem, leaf, and rhizome tissues of M. × giganteus sampled throughout the growing season (May to October) over 3 years revealed high concentrations in the spring rhizome, low levels in all tissues during the summer period of rapid growth, followed by increasing accumulation in stem and rhizomes after flowering. Elevated asparagine levels mark periods of active nitrogen remobilization from rhizome to shoot in spring, and from the shoot to rhizome in autumn. Fig. 4: Seasonal gene expression changes in miscanthus. a Shows asparagine in rhizome, stem, and leaves over the growing seasons normalized to total nitrogen in the sample. The error bars represent the standard deviation. b Principal component analysis of RNA-seq read counts normalized using the DESeq2 variance-stabilizing transformation method. PC1/2 distinguishes the three tissues from each other. c PC3/PC4 separates samples based on their nutrient mobilization status. The color scheme for the organs and dates matches b . d Heatmap across all tissues in the study comparing the expression of a subset of genes expressed in tissues that are actively remobilizing nutrients. Source Data are provided as a Source Data file. Full size image To characterize the seasonal dynamics of gene expression and regulatory programs associated with perenniality in Miscanthus , we performed RNA-seq from the same tissue samples collected for profiling nitrogen cycling (Supplementary Note 8 and Supplementary Data 1 ). Principal component analysis (PCA) identified the two largest sources of variation as tissue type, followed by sampling time (Fig. 4b ). Comparisons among tissues produced a catalog of organ-preferred genes (Supplementary Fig. 8 and Supplementary Data 1 – 9 ). As expected, leaf-preferred genes are significantly enriched in genes functioning in carbon fixation and metabolism, and stem-preferred genes include those associated with phenylpropanoid biosynthesis and amino acid metabolism. Gene expression in rhizomes is more similar to stems than leaves, consistent with their developmental origin as modified stems (Supplementary Fig. 8a, b ). Relative to stems and leaves, rhizomes preferentially express transcription factors that regulate growth and metabolic processes, and genes that respond to stimuli such as water and stress (Supplementary Fig. 8e ). We identified 35 genes that are preferentially expressed in the rhizome, including homologs of genes like GIANT KILLER ( GIK ) and SHORT INTERNODE ( SHI ) implicated in organ patterning, differentiation, and cell elongation [33] , [34] , [35] , [36] . Overexpression of SHI -like genes results in compact plants with shorter stem internodes [37] , [38] , [39] , which is consistent with the morphological differences between miscanthus rhizomes and stems. We identified and characterized the transcriptional network regulating seasonal nutrient mobilization in miscanthus (Supplementary Note 8 ), which is central to the perennial lifecycle and efficient recycling of resources. Although tissue identity dominates the first two principal components of gene expression, the third component (PC3) separates the spring rhizomes, fall leaves, and fall stems from the other tissues (Fig. 4c ). Differentially expressed genes contributing to the pattern in PC3 (Supplementary Note 8 ) comprise a dynamic network differentiating the fall rhizome that is storing nitrogen from the spring rhizomes that are releasing nitrogen to promote new growth (Supplementary Data 1 ). Of these genes, 104 had a functional or KEGG assignment, including a suite of transcription factors and genes with known important roles in nitrogen mobilization [40] like ASPARAGINE SYNTHETASE ( ASN1 ), GLUTAMATE DEHYDROGENASE ( GDH2 ), and GLUTAMATE DECARBOXYLASE ( GAD1 ). Remarkably, the most prominent (“hubby” or central) transcription factors within the network are a subset of JASMONATE ZIM DOMAIN (JAZ) family proteins that regulate jasmonic acid biosynthesis (e.g., ALLENE OXIDE SYNTHASE, AOS) and signaling, a pathway recently shown to activate nitrogen remobilization in rice [41] (Fig. 4d ). 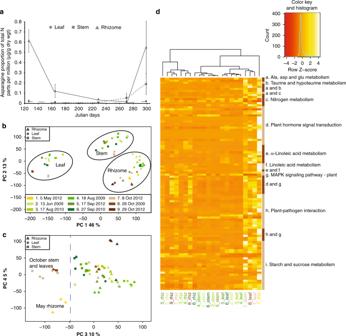Fig. 4: Seasonal gene expression changes in miscanthus. aShows asparagine in rhizome, stem, and leaves over the growing seasons normalized to total nitrogen in the sample. The error bars represent the standard deviation.bPrincipal component analysis of RNA-seq read counts normalized using the DESeq2 variance-stabilizing transformation method. PC1/2 distinguishes the three tissues from each other.cPC3/PC4 separates samples based on their nutrient mobilization status. The color scheme for the organs and dates matchesb.dHeatmap across all tissues in the study comparing the expression of a subset of genes expressed in tissues that are actively remobilizing nutrients. Source Data are provided as a Source Data file. These data reveal a group of regulators and enzymes that may be key for promoting the nitrogen remobilization in spring. Inter- and intraspecific variation and introgression Breeding to improve miscanthus for biomass and other applications can draw upon extensive wild germplasm from multiple species and ploidy levels. We therefore investigated the genetic diversity of Miscanthus and the distribution of inter- and intraspecific variation in admixed populations. We combined new WGS sequencing of 18 accessions of varying ploidy, including the triploid biofuel cultivar M . × giganteus “Illinois” (see Supplementary Note 9 and Supplementary Table 9 ) with previously generated genotyping-by-sequencing data from primarily wild accessions with broad geographic coverage [11] , [12] , [42] , [43] , spanning the native range of miscanthus across north- and south-east China, Korea, Russia, and Japan. Genome-wide admixture (Fig. 5a ) and PCA (Fig. 5b ) readily differentiate two species, M. sinensis and M. sacchariflorus . Other named Miscanthus accessions, such M . transmorrisonensis and M. floridulus , lie within the range of genetic variation of M. sinensis , suggesting that these taxa should more properly be considered subtypes of M. sinensis . The accession in our collection named Miscanthus junceus , however, is clearly distinct and appears to be more closely related to sugarcanes than Miscanthus (Supplementary Fig. 9 ). It is African, sometimes classified in a separate genus Miscanthidium , and clearly separate from Miscanthus sensu stricto [44] . Fig. 5: Miscanthus population structure and segmental ancestry. a Population structure of 407 miscanthus accessions, including 57 M . × giganteus , 120 M. sacchariflorus ( Msa ), and M. sinensis ( Msi ) from China (75), Korea (15), and Japan (140). b Principal component analysis of 407 miscanthus accessions where “x” marks admixtures of Msa and Msi . Such hybrids are collectively referred to as M . × giganteus (Mxg), and can be diploid, triploid, or tetraploid. Separation of Japanese and mainland Asian populations is largely consistent with structure analysis in a . Whole-genome shotgun (WGS)-sequenced accessions are labeled. c Segmental ancestry of miscanthus accessions based on WGS sequencing. Each horizontal bar denotes one (imputed) haploid chromosome set; red and blue indicate Msa and Msi ancestry, respectively. The number of bars represents ploidy. Introgression of M. sacchariflorus into M. sinensis (MsiEF148, Undine, DH2, DH2P) is common among cultivated European types (Supplementary Fig. 10 ). Source Data underlying Fig. 5c are provided as a Source Data file. Full size image Our chromosome-scale genome assembly allows us to investigate patterns of admixture in interspecific hybrids (Fig. 5c ). While all M. sinensis × M. sacchariflorus hybrids and admixtures are taxonomically characterized as M . × giganteus , this nothospecies has rich diversity due to the occurrence of diploid, triploid, and tetraploid accessions (Supplementary Fig. 10 ). We find that many ornamental diploids, especially many bred by Ernst Pagels in Germany, contain chromosomal segments of M. sacchariflorus introgressed into an M. sinensis background, consistent with prior admixture studies [11] , [12] . Mainland Asian and Japanese M. sinensis are distinct subpopulations (Fig. 5a ) that diverged ~500,000–1000,000 years ago based on chloroplast DNA (Supplementary Note 9 ). Our data confirm that the highly productive triploid biofuel M . × giganteus genotype, “Illinois,” is an interspecific hybrid of tetraploid M. sacchariflorus and diploid M. sinensis [14] , [45] . We find a predominant 2:1 ratio of M. sacchariflorus : M. sinensis alleles across the entire genome, consistent with this hypothesis; however, we also observed that the M. sacchariflorus ancestor had interspecific admixture (Fig. 5c and Supplementary Fig. 10c, e ), which indicates that the most productive miscanthus genotype currently grown is the product of more than one cycle of introgression from M. sinensis into M. sacchariflorus . Hybrids between M. sacchariflorus and M. sinensis are frequently highly vigorous and high-yielding, regardless of whether they are diploid, triploid, or tetraploid [46] , [47] . Thus, understanding how prior introgression of M. sinensis alleles into a primarily M. sacchariflorus genetic background affects the yield potential of subsequent interspecific hybrids will be important for optimizing breeding strategies. In particular, M . × giganteus combines the tufted habit (many stems per area; short rhizomes) of its M. sinensis parent with the spreading rhizomatous habit (few stems per area; long rhizomes) of its M. sacchariflorus parent, typically in an intermediate form, and optimizing the number of stems per area is critical to breeding for high yield in M . × giganteus [48] . The recently collected Japanese M . × giganteus triploid [49] “Ogi80” has a similar pattern to “Illinois,” with both including several short blocks containing two or three M. sinensis alleles. These regions could be due to segmental gene conversion or loss during the propagation of this sterile triploid, or interspecific introgression prior to triploid formation. Another natural triploid, “Ogi63,” shows a distinct pattern, highlighting the diversity of natural polyploid Miscanthus hybrids (Supplementary Fig. 10 ). Miscanthus is a promising perennial biomass source and candidate biofuel crop with efficient C4 photosynthesis that is highly adaptable. Its ability to grow on marginal lands with limited inputs, and its high drought and chilling tolerance make it suitable for both tropical and temperate climates. The genome sequence and genomic analysis presented here provides a foundation for systematic improvement of Miscanthus to optimize its productivity and robustness. Comparative analyses among the Andropogoneae [50] , which unites miscanthus with maize, sorghum, and sugarcane, promise to reveal the genetic basis for innovations that contribute to the high productivity and wide adaptation of this tribe of grasses. Genome sequencing and chromosomal assembly We shotgun-sequenced the M. sinensis genome at ~90× redundancy with Illumina paired-end and mate-pair data, augmented by fosmid-end pairs and in vitro and in vivo chromatin conformation capture (HiC) as described in Supplementary Note 1 . Illumina shotgun assembly was performed with Meraculous2 [51] and organized into chromosomes with HiC data using HiRise (Dovetail Genomics, Scotts Valley, CA) followed by manual curation with Juicebox [52] , and confirmation of internal self-consistency as described in Supplementary Note 2 . The assembly was further corroborated and assigned to chromosomes using a genetic map derived from four crosses, with 4298 uniquely assignable 64-bp markers, as described in Supplementary Note 3 . Protein-coding gene and transposable element annotation Protein-coding gene structures were annotated using the DOE Joint Genome Institute annotation pipeline [53] that incorporates transcriptional evidence, homology support from related grasses, and ab initio methods, as described in Supplementary Note 4 . RNA-seq data from three tissues and 57 timepoints for M . × giganteus and M. sinensis DH1 leaf and rhizome (PRJNA575573, SRP017791) were used, and these data are summarized in Supplementary Note 8 including accession numbers. Genome completeness was estimated using BUSCO [54] , and orthologous gene families identified using OrthoVenn [55] as described in Supplementary Note 4 . Transposable elements were identified de novo using RepeatModeler [56] to augment existing catalogs of grass repeats from repbase [57] and MIPS [58] using RepeatMasker [59] , and identified intact retrotransposons with LTRHarvest [60] , as described in Supplementary Note 5 . LTR families were defined by clustering these LTRs with those of sorghum and sugarcane by BLAST score using 90% identity and 90% length cutoffs as described in Supplementary Note 5 . Subgenome and homeologous exchange identification We partitioned the M. sinensis genome into subgenomes A and B by a modification of methods described in Session et al. [24] and described more fully in Supplementary Note 6 . Importantly, this method can be applied without requiring sequences from extant A and B diploids. Briefly, we identified 1187 13-bp sequences (13-mers) that (1) occurred at least 100 times across the genome, and (2) were at least twofold enriched in one member of each homeologous chromosome pair (excluding the case of fused homeologs). 13-mers were counted using Jellyfish [61] . Homeologous chromosomes were determined based on conserved synteny to each other and to sorghum (Fig. 1 ). These 13-mers allowed chromosomes to be clustered by subgenome, and were found to overlap with subgenome-specific repeats as described in Supplementary Note 6 . To identify cases of homeologous exchanges, we sought chromosomal regions whose 13-mer identity differed from the overall identify of the chromosome, using a hidden Markov model whose observed state was the number of A- and B-specific 13-mers and whose emitted state is A or B, as described in Supplementary Note 6 . Determination of biases in subgenome gene retention We used two methods to determine orthology between M. sinensis genes and sorghum in order to assess differential retention of gene duplicates after allotetraploidy, using sorghum as the outgroup representing the ancestral (preduplicated state). For the first method, gene families were constructed using OrthoVenn [55] . For the second method, we used BLAST-based clustering. Subgenome-specific retention is defined as the number of genes on a given subgenome divided by the number of inferred ancestral (i.e., preduplication) gene number. Details of this analysis can be found in Supplementary Note 6 . Timing of events associated with allotetraploidy We estimated the timing of speciations in the Andropogoneae using a set of 1:1 orthologs for species shown in Fig. 1c with P. hallii and S. italica as outgroups, as described in Supplementary Note 7 . Briefly, concatenated multiple-sequence alignments were produced using Dialign-TX [62] and Gblocks [63] . M. sinensis and maize genes were partitioned into A and B subgenomes, and 1 and 2 subgenomes, respectively, with 1–2 assignments as determined by Schnable et al. [28] . The dataset included M. sacchariflorus A and B genes predicted by mapping diploid M. sacchariflorus shotgun sequence to the M. sinensis assembly. M. sacchariflorus has the same karyotype as M. sinensis , and hybrids are fertile, indicating that they share the same A/B ancestral tetraploidy. Phylogenies were produced from the resulting 28,887 nucleotide alignment using PhyML [64] . Timetrees were estimated using r8s [65] with a smoothing parameter of 0.1, and constraining the Setaria / Panicum node to 12.8–20 Mya and the Sorghum /maize split to 13–21.2 Mya [66] . We estimated the period during which the A and B progenitors were separate species using phylogenies of five subgenome-specific LTR families with ≥100 members that contain a subgenome-enriched 13-mer, as described in Supplementary Note 7 . Subgenome-specific LTR families have been active when the two progenitors were separate species, but before allotetraploidy. To calibrate the rate of LTR substitution in miscanthus, we used LTR families that are (1) found in high copy number in miscanthus across both the A and B subgenomes, and so were active after allotetraploidy, and (2) have parallel activity in the sorghum genome, and used a miscanthus–sorghum divergence time of 10 My as determined from protein-coding genes. We used the median substitution rate of these families (2.1 × 10 −8 substitutions per My) to infer the timing of subgenome-specific activity based on Jukes–Cantor distance. Details are provided in Supplementary Note 7 . Analysis of gene expression We analyzed RNA-seq data using Tophat2.1.1 [67] , HTSeq [68] , DESeq2 [69] , and the NOISeq R package [70] , [71] to extract expression levels and further analyze the RNA-seq data as described in Supplementary Note 8 . To identify genes that were constitutively expressed in any one organ type, we considered only genes with a count per million (cpm) of 5 or greater within all samples of an organ type. KEGG enrichment analysis using keggseq [72] was performed on genes that were preferentially in leaves, stems, and rhizomes, respectively, to determine if they clustered into specific pathways or functional categories. Enriched pathways with a q value ≤ 0.01 are shown in Supplementary Fig. 8c–e . For the purposes of comparing gene expression of homeologs, we measured gene expression using cpm, after combining replicates, as described in Supplementary Note 8 . In order to measure subgenome expression bias, for each homeolog pair, we considered only experiments where one or both homeologs have nonzero expression (cpm > 0.5). This condition is necessary because the majority of genes are not expressed in every tissue, leading to a large number of uninformative comparisons. We considered expression bias using a variant of the approach of Schnable et al. [28] , identifying homeolog pairs where one member of the pair was expressed X -fold relative to the other, where X = 2, 5, and 10, again requiring both members to be expressed at a minimal level (cpm > 0.5) to avoid uninformative comparisons. Analysis of genetic variation WGS sequences of 18 miscanthus accessions (Supplementary Table 9 ) were aligned to the haploid M. sinensis DH1 reference sequence using bwa mem [73] , and variants called using GATK [74] version 3.6, as described in Supplementary Note 9 . Restriction site-associated DNA-sequencing (RAD-seq) data from 2819 Miscanthus individuals were used to obtain a snapshot of genetic diversity, as described in Supplementary Note 9 . For PCA with the RAD-seq data genotypes, we retained SNPs with a maximum of 30% missing data and a minimum minor allele frequency of 0.01, resulting in a set of 144,337 SNPs. From this dataset, individuals with 50% or more missing data were removed, leaving 2492 out of the original 2819 individuals. By filtering SNPs and individuals in this way, the remaining data were primarily derived from Pst I sequencing libraries, as this was the enzyme most commonly used across the dataset. Genotypes were coded on a numeric scale from 0 to 1, indicating copy number for the nonreference allele, i.e., 0, 0.5, and 1 for diploids, 0. 0.33, 0.67, and 1 for triploids, and 0, 0.25, 0.5, 0.75, and 1 for tetraploids. PCA was performed using probabilistic PCA method implemented in the Bioconductor package pcaMethods [75] . All SNPs were centered and scaled to unit variance before PCA. The genomic makeup of the accessions was analyzed with ADMIXTURE [76] . 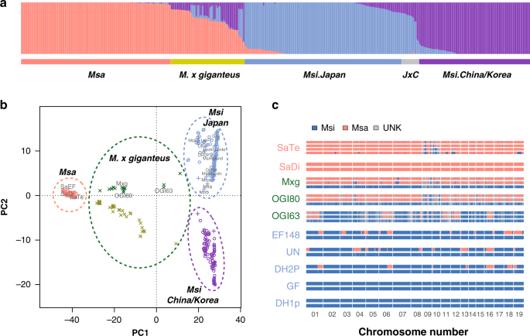Fig. 5:Miscanthuspopulation structure and segmental ancestry. aPopulation structure of 407 miscanthus accessions, including 57M. ×giganteus, 120M. sacchariflorus(Msa), andM. sinensis(Msi) from China (75), Korea (15), and Japan (140).bPrincipal component analysis of 407 miscanthus accessions where “x” marks admixtures ofMsaandMsi. Such hybrids are collectively referred to asM. ×giganteus(Mxg), and can be diploid, triploid, or tetraploid. Separation of Japanese and mainland Asian populations is largely consistent with structure analysis ina. Whole-genome shotgun (WGS)-sequenced accessions are labeled.cSegmental ancestry of miscanthus accessions based on WGS sequencing. Each horizontal bar denotes one (imputed) haploid chromosome set; red and blue indicateMsaandMsiancestry, respectively. The number of bars represents ploidy. Introgression ofM. sacchariflorusintoM. sinensis(MsiEF148, Undine, DH2, DH2P) is common among cultivated European types (Supplementary Fig.10). Source Data underlying Fig. 5c are provided as a Source Data file. Figure 5a shows the result for K = 3, which was used to analyze the populations. To resolve admixture along chromosomes, we identified 1283,756 species-specific SNPs in the nonrepetitive regions of 19 chromosomes from fixed differences between the two species as represented by 4 diploid exemplar genomes without evident admixture as described in Supplementary Note 9 . These ancestry-informative markers were used to obtain a high-resolution admixture map for the WGS accessions (Fig. 5c ), following the method of Wu et al. [77] . A subset of these ancestry-informative markers that overlapped RAD-seq variants were used to infer the segmental ancestry of the RAD-seq accessions. Further details are provided in Supplementary Note 9 and Supplementary Data 10 . Reporting summary Further information on research design is available in the Nature Research Reporting Summary linked to this article.